An intuitive and efficient method for cell voltage prediction of lithium and sodium-ion batteries The voltage delivered by rechargeable Lithium- and Sodium-ion batteries is a key parameter to qualify the device as promising for future applications. Here we report a new formulation of the cell voltage in terms of chemically intuitive quantities that can be rapidly and quantitatively evaluated from the alkaliated crystal structure with no need of first-principles calculations. The model, which is here validated on a wide series of existing cathode materials, provides new insights into the physical and chemical features of a crystal structure that influence the material potential. In particular, we show that disordered materials with cationic intermixing must exhibit higher potentials than their ordered homologues. The present method is utilizable by any solid-state chemist, is fully predictive and allows rapid assessement of material potentials, thus opening new directions for the challenging project of material design in rechargeable batteries. Over the past 20 years, intensive research has been devoted to the design of new promising materials for positive electrodes in Li-ion batteries [1] , [2] , [3] , [4] . The candidates have to be safe, cheap and environmentally friendly along with exhibiting high energy density and good rate capability. Beside the economic and ecologic aspects on which chemists can act to meet the industrial specifications of ideal materials, fundamental chemistry can also be used to improve the electrochemical performances of electrodes in terms of energy density. In principle, the battery energy density should not be difficult to control (that is, improve) as it depends on two thermodynamic quantities—the specific capacity C (mAh g −1 ) and the working voltage E (Volt)—which are both fundamentally understood and therefore easily tunable. In practice, however, the literature teaches us that these two quantities are not so easy to improve simultaneously. In this context, high-throughput calculations and more generally combinatory approaches have emerged in the literature to scan a wide variety of materials and guide experimentalists in their search for high performance electrode materials [5] , [6] . Based on various techniques to sample the energy landscape of a periodic material, these approaches are very powerful to predict the most stable crystal structure for a given chemical composition. However, in the case of electrode materials neither the voltage nor the capacity are functional of one given composition, that is, the link between one material structure/energy and its electrochemical performance is not direct. So far, within the Density Functional Theory (DFT) framework, the calculation of a material potential requires the computation of accurate reaction enthalpies [7] . Although this may appear much easier to conduct than experiments, the procedure still requires a significant amount of work: both the alkali-rich and the alkali-poor compositions have to be computed within a reasonable numerical accuracy for their energy difference to be meaningful, and sometimes with functionals that go beyond the usual local density approximation [8] or generalized gradient approximation [9] , [10] . While this is certainly tractable for a quite large set of compounds [5] , [11] , it becomes limited or prohibitive when realistic materials including defects, disorder or dopants must be studied [12] , [13] . Above all, first-principles calculations are not straightforwardly utilizable by non informed users. To overcome these limitations and provide an efficient and affordable tool to experimentalists to evaluate material potentials, a direct link between some of the material properties and the operating cell voltage of the battery is strongly needed. This implies understanding which and how the different constituents of a material contribute to the amplitude of the potential, that is, how the electronic structure of the material is linked to the intrinsic nature of its constituting elements and to the way they interact all together in the crystal. A step towards this direction was done in the study by Goodenough and co-workers [14] , [15] who correlated the nature of the Metal–Ligand ( M − L ) bonds to the material potential, through the so-called inductive effect. This qualitative approach has been largely validated with the successful development of a tremendous variety of high-potential transition metal ( M ) polyanionic systems. Among them, the famous olivine LiFePO 4 (ref. 14 ) and the more recent triplite LiFeSO 4 F (refs 16 , 17 ) exhibit potentials versus Li + /Li 0 (the counter electrode currently used in laboratory half-cells) as high as 3.45 V and 3.9 V, respectively, compared with <3 V for standard Fe-based oxides. Although very powerful, this approach is also perfectible in particular to address the polymorphism issue recently raised by the LiFeSO 4 F tavorite versus triplite polymorphs whose potentials versus lithium are 3.6 V and 3.9 V, respectively, despite equivalent inductive ligands [16] , [18] . In this paper, we propose a general approach to discriminate the role of the transition metal, the ligands, the crystal structure and the alkali stoichiometry on the voltage amplitude. This is achieved through the formal writing of the cell voltage into meaningful quantities, which are also numerically accessible at a modest cost, that is, free of any DFT calculations. We demonstrate that the potential of cathode materials is linked to the site energies of the added A + /e − species ( A =Li, Na). It accounts not only for the short-range inductive effect of the ligands onto the transition metal redox energy, but also for an additional electrostatic term coming from the screening effect of the Li + ions into the material structure. The latter can be seen as an electrostatic stabilization of the negatively charged host material and gives rationale to the first-order contribution of the Li + ions to the cell voltage of electrode materials, which, in turn, provides clear insights into the origin of potential variations in various polymorphs. The cell voltage decomposes into one on-site contribution directly linked to the chemical potential and chemical hardness of the redox-active centre (RAC) and two inter-site electrostatic contributions due to the A + and e − added charges. In the specific case of strongly ionic systems, these terms reduce to two Madelung contributions that can be rapidly evaluated using simple formal punctual charges that are very familiar to chemists, and which linearly correlate with the battery cell voltage. This new formulation not only discards the two-step DFT procedure required so far to accurately compute cell voltages but is also valid for any crystal structure, any ligand, any transition metal and any alkali type and stoichiometry. It also provides with a tractable treatment of disorder such as A / M (alkali/transition metal) intermixing whose effect is here demonstrated to substantially increase the material potential compared with ordered materials displaying equivalent ligand field. Owing to its generalized expansion into meaningful and easily tunable quantities, our approach provides solid-state chemists new recipes for designing new electrode materials for Li-ion (or Na-ion) batteries. In the future, it can also be coupled to crystallographic databases (such as the ICSD [19] , [20] or COD [21] , [22] , [23] ) to rapidly estimate the potentials of a wide variety of compounds, thus allowing a powerful sampling of the most promising candidates for A -ion ( A =Li, Na) battery materials. General formulation The derivation of the battery cell voltage necessitates to begin with the reversible reactions occurring at the positive (high potential versus A + / A 0 ) and negative (low potential versus A + / A 0 ) electrodes in a current electrochemical cell. During the charging and discharging of an alkali-ion battery, A + ions and electrons are exchanged between the positive and the negative electrodes. When the A 0 metallic electrode is used as the reference negative electrode, the overall reaction corresponds to a variation in the alkali chemical composition of the intercalation material used at the positive electrode, hereafter named the host material (Host). The distribution of the added charges ( A + and electrons) into the host material obviously differs from that of the reference metallic electrode and depends on the electronic structure of the host material, that is, whether the electrons are localized or delocalized in the system. The difference in the A + /e − charge separation between the two electrode materials depends on their respective Galvani potentials and is at the origin of the cell voltage amplitude. To investigate the contribution of each charged species to the battery voltage, it is convenient to introduce an additional step in the overall electrochemical reaction, which corresponds to the formation of a virtual phase (hereafter denoted A ⊕ ⊖ ) in which the alkali ions (refered to as ⊕ ) and the electrons (refered to as ⊖ ) are distributed as in the A -rich material. This is illustrated on the schematic picture of Fig. 1 where the host material unit cell is represented by a positively charged transition metal surrounded by its negatively charged ligands and where the formation energy of the A -rich material can be seen as the interaction energy between the A -poor material and the virtual phase. The overall thermodynamic reaction is here assumed to be solvent-independent [24] , thus decomposing into four different steps, each associated with a well-defined reaction energy. 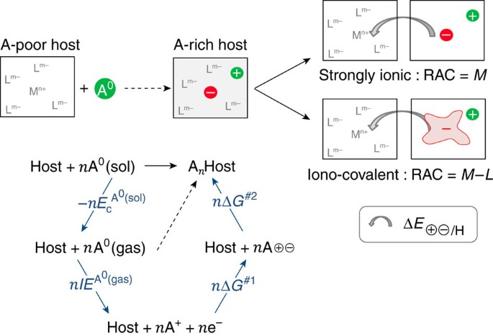Figure 1: Charge separation in the alkaliated phase. Illustration of the electrochemical transformation of theA-poor host material into theA-rich material through the reaction with the alkali and solvent-independent decomposition of the overall reaction into four sub-reactions. The host material is represented as positively chargedMn+surrounded by negatively charged ligandsLm−, while the added alkali ions (A+) and electrons (e−) are illustrated by red and green circles, respectively. Depending on the nature of the redox-active centre (RAC) the electrons localize either on the transition metal or on theM−Lbonds.,and ΔG#1−2refer to the sublimation energy ofA0(sol) intoA0(gas), the ionization energy ofA0(gas) into isolatedA+and e−species and the reaction energy to form the virtual phaseA⊕⊖and the alkaliated hostAnHost. Figure 1: Charge separation in the alkaliated phase. Illustration of the electrochemical transformation of the A -poor host material into the A -rich material through the reaction with the alkali and solvent-independent decomposition of the overall reaction into four sub-reactions. The host material is represented as positively charged M n + surrounded by negatively charged ligands L m − , while the added alkali ions ( A + ) and electrons (e − ) are illustrated by red and green circles, respectively. Depending on the nature of the redox-active centre (RAC) the electrons localize either on the transition metal or on the M − L bonds. , and Δ G #1−2 refer to the sublimation energy of A 0 (sol) into A 0 (gas), the ionization energy of A 0 (gas) into isolated A + and e − species and the reaction energy to form the virtual phase A ⊕ ⊖ and the alkaliated host A n Host. Full size image At equilibrium and constant pressure and temperature, the open-circuit cell voltage, V cell is linked to the reaction Gibbs energy of the overall process (Δ r G T , p ) through the Nernst equation: where μ i are the chemical potentials of the bulk and gas phases and represents the chemical potential of the counter electrode (metallic alkali). and are the ionization energy of the alkali atom and the sublimation energy of the A 0 (sol) alkali metallic phase (that is, cohesive energy), respectively. Δ G #1 is the formation energy of the virtual phase from the isolated A + and e − charged species, whose chemical potentials are perfectly defined through the ionization of the A 0 (gas) gas phase. Δ G #2 is simply the formation of the A -rich phase from the A -poor and the virtual phases. Before evaluating these two terms, it is interesting to show how they are linked to the RAC of the electrochemical reaction that is, on the nature of the chemical bonds in the host material. In transition metal-based ionic systems such as high-potential cathode materials, the bands involved in the redox process of the electrochemical reaction can be easily deduced from the molecular orbitals (MOs) of the ML n redox entity. Within an orbital approach to the ligand field, the effective interaction β M − L between a transition metal ion (positively charged) and its surrounding ligands (negatively charged) is proportional to S 2 /Δ χ , where S is the overlap between the interacting metallic d -orbitals and ligands s , p -orbitals, and Δ χ the electronegative character of the ligands with respect to the transition metal. The effective β M − L interaction then sets the relative weight of the transition metal ( C M ) and ligand ( C L ) atomic orbitals into the bonding ( ψ ) and antibonding ( ψ *) MOs. The antibonding MOs, which are closer in energy to the metallic d -orbitals, are characterized by while the bonding MOs which are closer in energy to the ligand s , p -orbitals are characterized by . As shown in Fig. 2 , β M − L decreases with both the increase of the electronegative character of the ( XO 4 ) n − ligand and the polarization of the O(2 p ) towards the tetrahedral X coordination sphere, thus decreasing C L in ψ * and C M in ψ . Because the bands involved in the redox process, that is, those accommodating the added electron upon reduction, mainly come from the ψ * electronic levels, the ligand participation to the electrochemical reaction directly depends on the C L weight in ψ *, which also defines the RAC. As shown in the schematic picture of Fig. 3 , the added electron either partially delocalizes over the M − L bonds (RAC= M − L ) in case of actor ligands ( C L ≠0) or fully localizes on the transition metal (RAC= M ) in case of spectator ligands ( C L →0). The latter is the ‘free-ion’ limit for which the inductive effect is so high that the redox energy of the RAC+e − →RAC − electronic reduction (namely μ RAC/RAC −) tends to the redox couple of the solvated ion accessible in current handbooks of physical chemistry. In that case, the M charge or equivalently the Madelung field experienced by the transition metal in its ligand field is a direct measure of the ligand inductive effect (that is, the ligand participation to the redox process, C L ). As illustrated in Fig. 3 , the Madelung field computed at the M site using first-principles DFT Bader charges on a wide series of iron-based polyanionic systems clearly discriminates different classes of ligands (see Supplementary Tables I and II and Supplementary References for details). Nevertheless, it shows only a poor correlation with the experimental open-circuit voltages of these systems and cannot be considered as a quantitative and accurate measure of the materials potential. To achieve a quantitative model, it is then necessary to evaluate the areformentioned Δ G #1 and Δ G #2 in the general case where no a priori assumption is made on the ligand contribution to the redox property of the material and where a full electron transfer is assumed from the alkali to the RAC ( q ( q ⊕ )=− q (− q ⊖ )=1). 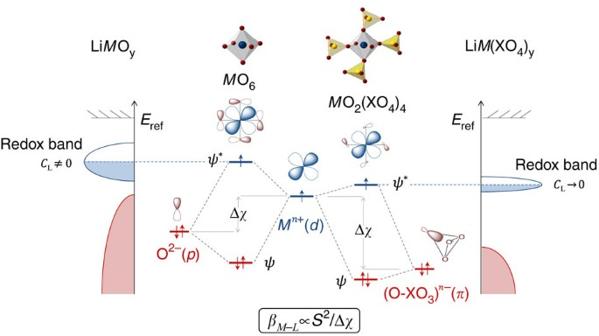Figure 2: Schematic density of states of transition metal oxides and transition metal polyanionic systems as deduced from local orbital interactions. Illustration of the effective local interactionβM−Lbetween the metallicd-orbitals and the ligandsp-orbitals as a function of the electronegative character of the ligand with respect to the transition metal (Δχ) and its consequence on the ligand participation to the electronic density of states and redox activity of the material.ψandψ* are the bonding and antibonding molecular orbitals of theMLnredox entity andCLreflects the weight of the ligandsp-orbitals into the redox band of the material. For sake of clarity, only oneM(d) orbital is represented and not split by the Mott gap, as expected in strongly correlated systems. Figure 2: Schematic density of states of transition metal oxides and transition metal polyanionic systems as deduced from local orbital interactions. Illustration of the effective local interaction β M − L between the metallic d -orbitals and the ligands p -orbitals as a function of the electronegative character of the ligand with respect to the transition metal (Δ χ ) and its consequence on the ligand participation to the electronic density of states and redox activity of the material. ψ and ψ * are the bonding and antibonding molecular orbitals of the ML n redox entity and C L reflects the weight of the ligands p -orbitals into the redox band of the material. For sake of clarity, only one M ( d ) orbital is represented and not split by the Mott gap, as expected in strongly correlated systems. 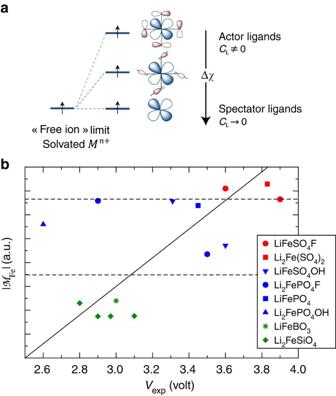Figure 3: Orbital picture of the ligand field effect and its consequence on the transition metal Madelung field. Illustration of the ligand inductive effect on the energy of the molecular orbitalsψ* involved in the redox activity of a material through theCLindicator, and its consequence on the Madelung field experienced by the transition metalin several lithiated Fe-based compounds (see Methods section for details of Madelung calculations).is here plotted with respect to the experimental open-circuit voltage (in abcisse). The horizontal lines discriminate the different classes of ligands, which are represented in different colours. Equivalent labels and colours correspond to different polymorphs of an equivalent chemical composition. Details for the crystal structures and experimental voltages of the tested phases are given inSupplementary Tables I and IIandSupplementary References. Full size image Figure 3: Orbital picture of the ligand field effect and its consequence on the transition metal Madelung field. Illustration of the ligand inductive effect on the energy of the molecular orbitals ψ * involved in the redox activity of a material through the C L indicator, and its consequence on the Madelung field experienced by the transition metal in several lithiated Fe-based compounds (see Methods section for details of Madelung calculations). is here plotted with respect to the experimental open-circuit voltage (in abcisse). The horizontal lines discriminate the different classes of ligands, which are represented in different colours. Equivalent labels and colours correspond to different polymorphs of an equivalent chemical composition. Details for the crystal structures and experimental voltages of the tested phases are given in Supplementary Tables I and II and Supplementary References . Full size image Δ G #1 corresponds to the condensation of the isolated charged species into the virtual phase and then restricts to their self-electrostatic interactions: where V ⊕ ⊖ ( r A ) and V ⊕ ⊖ ( r ) are the electrostatic fields experienced by the added charges in the virtual phase and ρ ⊖ ( r ) is the added electronic charge density. Because the latter may localize on the transition metal (RAC= M ) or delocalize over the M − L bonds (RAC= M − L ) the integral runs over the volume of the added electron density (see Fig. 1 for iono-covalent systems). Δ G #2 corresponds to the interaction energy between the A -poor phase and the virtual phase and can then be obtained following standard perturbation theory. Noteworthy, when the structural modifications induced in the host matrix by the electrochemical process are weak over the electronic perturbation due the added charges (which is generally the case in strongly ionic systems), solely the crystal structure of the A -rich phase is required to evaluate this reaction energy. In that case Δ G #2 restricts to a simple interaction energy, namely Δ E ⊕ ⊖ /H , which decomposes into one electronic and one ionic contribution: In this expression, V H ( r A ) and V H ( r ) are the electrostatic fields exerted by the charged M n + and L n − ions of the host matrix at the A and RAC sites, is the chemical potential of the RAC (assimilated to the Fermi level of the host material in Fig. 2 ) and η RAC is the chemical hardness of the RAC. Note that the term in parenthesis corresponds to the change in the RAC electronic levels with respect to their initial energy due to the variation of the number of electrons in the system ( δq ⊖ =1). Interestingly, this electronic contribution Δ E ⊖ /H is here decomposed into short-range and long-range interactions, that is, the on-site interaction of the added electron with the other electrons of the RAC and the inter-site electrostatic interactions with the surrounded charges of the host material. Rearranging equations (2) and (3) and introducing , then the open-circuit cell voltage with respect to the alkali reference becomes: where is a second-order (negligible) interaction energy avoiding double counting. This decomposition gives a novel formulation of the cell voltage of an A -ion battery into meaningful and tunable quantities. By dissecting the different factors controlling the material potential in terms of electronic versus ionic and short-range versus long-range contributions, it brings out which quantities are controlled by the RAC intrinsic nature ( M / L couple) or by the crystal structure (polymorph), therefore providing clear new directions to chemists for designing new materials. Electronic versus ionic contributions . Equation (4) shows that the cell voltage depends on one electronic and one ionic contribution: the former reflects the energy variation due to the electronic reduction of the host material H+e − →H − ; the latter reflects the change in the material Galvani potential due to the change in the material chemical composition. This ionic contribution is a first-order electrostatic contribution to the cell voltage and is therefore of great importance to understand the voltage variations observed in various polymorphs (equivalent chemical compositions but different M / A distributions) or in thermodynamically driven multi-step electrochemical reactions (different A -sites). Short-range versus long-range contributions . The cell voltage also gathers short-range and long-range effects. The two first terms of equation (4) are intrinsic to the RAC chemical nature and mainly short ranged. They include the ligand field effect though the ψ * orbital energy and the energy destabilization of ψ * due to the addition of an electron (2 η RAC ). The chemical hardness η RAC is a very important intrinsic property, which defines how the electronic levels of the system respond to an electronic reduction. It can be assimilated to the on-site U eff repulsion energy currently used by computational chemists in DFT+U calculations [25] to describe materials with strongly localized d - and f -electrons. Both quantities are linked in the conceptual DFT formalism [26] to the ionization potential (IP) and the electron affinity (EA) of a molecule or a solid through . Chemically speaking, the covalence of the M − L bonds (that is, the ligand participation to the Fermi level C L ) acts as a moderation of the transition metal chemical hardness η M exactly as it acts as a moderation of the U M values when going from M -based polyanions to oxides, sulphides, phosphides and so on. Because this on-site energy variation dominates over the inter-site energy variation (see below), the cell voltage will be as high as the electrode material is hard. This property can be easily tuned through the choice of the transition metal, its oxidation state and its surrounding ligands (see Fig. 2 ). Hence, provided that the pertinent electrochemical entity (RAC) is clearly defined, the macroscopic electrochemical property of a condensed phase can be deduced from microscopic quantities ( β M − L interactions), which are easily obtained from basic tight-binding approaches. In contrast, the two (non-negligible) other terms of equation (4) corresponds to the inter-site (long-range) electrostatic interactions of the added charges in the A -rich phase. They depend on the crystal structure of the insertion material and on the A -stoichiometry. Theses two quantities contribute to the cell voltage with opposite signs, showing that the loss of inter-site electrostatic interactions due to the addition of an electron is further balanced by a gain of inter-site electrostatic interactions due to the addition of the alkali ion. This demonstrates that, for one given M / L couple, the cell voltage should be as high as these inter-site electrostatic contributions are efficiently balanced. Noteworthy, in strongly ionic systems where the added electron is localized on the cationic transition metal sites, these contributions may cancel out when a 50:50 M / A intermixing occurs in the A -rich phase, that is, when both A and M are statistically and equally distributed over one given crystallographic site. Such disordered phases exist only at finite temperatures when the contribution of the configuration entropy to the free energy is higher than the formation energy of any ordered phase. This result is remarkable since disordered materials may also exhibit less ionic kinetic limitations than currently admitted, as recently shown in layered oxides [27] . In all other cases, including other x : y intermixing ratios resulting from the competition between finite temperature entropy and 0 K ordering stabilization, there is no reason to neglect these interactions, which are crucial to quantitatively reproduce the cell voltage of polymorphs. The ionic limit Focusing more specifically on strongly ionic systems, that is, systems having spectator ligands in Fig. 1 , the added electron localizes on the transition metal sites (RAC= M ) so that ρ ⊖ ( r ) can now be assimilated to a punctual negative charge q ⊖ . In that case tends to , that is, the redox energy of the solvated ion (‘free-ion’ limit). As mentioned above and previously stated by Goodenough and co-workers [15] following crystal field theory, this redox energy is directly proportional to the Madelung field experienced at the M sites in the A -rich phase . Adding the A + contribution which can also be evaluated by the Madelung field experienced at the A -sites in the A -rich phase the cell voltage of strongly ionic materials restricts to: The numerical application of this equation for a wide series of M -based polyanionic systems exhibiting different transition metal ( M =Fe, Co), different ligands, different A stoichiometries and different crystal structures is given in Fig. 4 , where the colours refer to the different classes of ligands deduced from Fig. 3 . A very good correlation is obtained between the theoretical and experimental cell voltages—even within the rough approximation of formal charges ( Fig. 4a ). Interestingly, the use of DFT Bader charges instead of simple formal charges does not significantly improve the results ( Fig. 4b ). This highlights that the variation of the metal charge from one polymorph to another has a negligible impact on the cell voltages of high-potential cathodes. 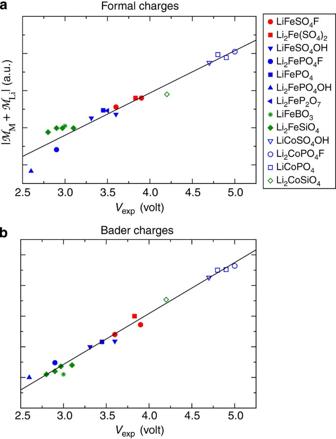Figure 4: Numerical application. Theoretical cell voltages for a series of Fe- (plain symbols) and Co-based (empty symbols) insertion materials estimated from equation (5) with (a) formal charges and (b) Bader charges obtained from first-principles DFT+U calculations (see Methods section for details). Figure 4: Numerical application. Theoretical cell voltages for a series of Fe- (plain symbols) and Co-based (empty symbols) insertion materials estimated from equation (5) with ( a ) formal charges and ( b ) Bader charges obtained from first-principles DFT+U calculations (see Methods section for details). Full size image The model described above gives new insights into the physical and chemical features of a crystal structure that influence a material potential, thus allowing to fully rationalize the origin of cell voltage variations from one system to another. Given that the neighbouring shell of the cationic sites are the negatively charged ligands, both and are negative and primarily dominated by the short-range Metal-Ligand (M-L) and A -Ligand ( A − L ) interactions. The latter is clearly a first-order effect, as confirmed by a simple comparison of Figs 3 and 4 , and contrasts with the recent statement by Melot et al. [28] of a so-called ‘secondary inductive effect’ of the alkali ions. In their work, these authors proposed that the number of A − L interactions in the A -rich phase should correlate with the cell voltage. While their assumption is intuitively fair, the way they further propose to capture this effect through the computation of the M atomic charge omits the first-order and dominant electrostatic contribution of the alkali metal, as expressed in equation (3). In his work on the Li x Mn 2 O 4 phases, Goodenough [2] also invoked the role of the Li-sites coordination to explain the 1 V shift in potential experimentally observed for this electrode material, which clearly corroborates the first-order contribution of the alkali ions. The potentials of the contentious LiFeSO 4 F tavorite (3.6 V) and disordered triplite, (3.9 V) polymorphs [12] , [16] , [17] , [18] are well-reproduced by our model (see red plain circles in Fig. 4 ). Since the Madelung field on the iron site is roughly equivalent for the two polymorphs (see Fig. 3 ), the origin of the jump of potential between the tavorite and the triplite is clearly attributed to the Li + contribution (see Fig. 4 ). The disorder in the triplite LiFeSO 4 F is characterized by a 50:50 M / A intermixing, while both cations lie on different crystallographic sites in the tavorite LiFeSO 4 F. As shown in the previous section, the inter-site electrostatic contributions cancel out in this case so that the cell voltage is dictated by the on-site contributions, namely and η RAC . Because both the tavorite and triplite polymorphs have nearly equivalent on-site contributions (that is, RAC= M in both cases), the potential of the disordered triplite polymorph is expected to be higher than the potential of any of its ordered homologues, which is well-reproduced by our model. The statistical distribution of the triplite polymorph is here fully accounted in our Madelung calculations through the use of averaged +1.5 formal charges on the cationic sites, while the ordered distribution of the tavorite polymorph is treated as punctual +2 and +1 charges. This can be systematically done for any type of inter-mixed or disordered materials (for example, LiFeP 2 O 7 ; (ref. 29 )). Such result is of particular importance since periodic DFT calculations are unable to account for a statistical distribution of charges, therefore avoiding accurate potential predictions for disordered materials (see Supplementary Fig. 1 ). In the same line, the layered LiFeSO 4 OH (3.6 V; (ref. 30 )) and the tavorite-like LiFeSO 4 OH (3.3 V; (ref. 31 )) also show a 0.3 V jump of potential despite equivalent ligands (see blue plain down triangles in Fig. 4 ). In contrast to the previous case, no Li/Fe intermixing occurs in the high-potential phase. The higher potential of the layered LiFeSO 4 OH is once again correlated to the crystal structure through the inter-site electrostatic interactions: on one hand, strong Fe-Fe repulsive interactions occur as the result of face-shared FeO 4 (OH) 2 octahedra [32] . This decreases the amplitude of in this layered polymorph compared with the tavorite-like polymorph (see Fig. 3 ). On the other hand, some oxygen atoms in the layered structure are not bonded to the iron, leading to dangling S–O bonds, which are much more efficiently screened by the Li + added charges. This substantially increases the amplitude of the , leading to a higher cell voltage. Another interesting scenario to highlight is the comparison of equivalent crystal structures having different ligands. For instance, the tavorite Li 2 FePO 4 F (2.9 V, blue plain circles) versus tavorite-LiFeSO 4 OH (3.3 V, blue plain down triangle) versus tavorite LiFeSO 4 F (3.6 V, red plain circle). Given that (PO 4 ) 3− is less inductive than (SO 4 ) 2− , the lower potential of the former is quite obvious. In addition, the OH − group is less electronegative than the F − ligand, which also explains the 0.3 V difference between the two latter. However, the ligand field cannot itself explain a 0.7 V difference between the Li 2 FePO 4 F and LiFeSO 4 F potentials. This time, the Li-stoichiometry is responsible for such a large potential difference. The amplitude is clearly much lower in Li 2 FePO 4 F due to the increasing number of Li + –Li + repulsive interactions with the increase in Li-stoichiometry. This result is also important as it emphasizes that capacity increase should necessarily be detrimental to the potential. These examples highlight the significant contribution of the Li + ions to the cell voltage amplitude, which, in no way, can be considered as a secondary inductive effect. The nice correlation obtained in Fig. 4 between theory and experiment also shows that our model is robust to evaluate the cell voltage of high-potential cathodes with no other need than the crystal structure of the alkali-rich composition. This also allows avoiding time-consuming DFT reaction enthalpy calculations and their related methodological issues (for example, DFT functionals, U eff values and statistical distributions) to predict material potentials. To conclude, the model presented in this work is the first quantitative model, free of first-principles DFT calculations, allowing an accurate and non-parameterized evaluation of potential variations in cathode materials, with an excellent accuracy. Since the needed ingredients of the model require insignificant numerical cost and corresponds to easy-handling quantities that can be manipulated by any solid-state chemist, it is expected to accelerate significantly the discovery of new materials suitable for being used as electrodes in lithium- or sodium-ion batteries. For instance, it can be used by experimentalists as soon as they know the structure of the compound under investigation, or it can be coupled to large crystal structure databases to perform a systematic search. More fundamentally, the model dissects all the leading parameters governing the material potentials in terms of ionic versus electronic and short-range versus long-range effetcs, thus providing recipes going beyond the inductive effect to design new materials. It is theoretically valid for any cathode material for which the A + oxidation state can be assumed. Compared with the state-of-the-art periodic DFT calculations that fail to predict the potential of disordered materials, our model solves this issue thanks to the use of handy averaged formal charges. Furthermore, it addresses the polymorphism issue, which was lacking in the approach by Goodenough [14] by including the crystal structure contribution to the cell voltage. A straightforward extension of the model to anode materials will consider partial charge transfer between the lithium and the host material, leading to a A δ + / δ e − (0≤ δ <1) charge separation. Promising candidates for high potential should then combine low-lying redox levels (low ), highly inductive surrounding ligands (high Δ χ ) and intermixing M / A cationic sites (balanced electrostatic contributions due to the ⊕ and ⊖ added charges). While the two former are chemically tunable with appropriate chemistry, especially by chosing the proper M / L couple, the latter is linked to the crystal structure and is much difficult to control. Nevertheless, the number of synthetic routes developed so far for material fabrication gives hope that this perspective is reasonably conceivable. Madelung field calculations Madelung fields were computed with a home-made programme based on the method by Ewald [33] using either Bader charges as obtained from periodic DFT+U calculations or formal charges (O 2− , F − , Si 4+ , P 5+ , S 6+ , Fe 2+ , Co 2+ , Li + , (OH) − =O − H). For the tavorite-LiFeSO 4 OH and Li 2 FePO 4 F phases, for which no experimental crystal structure is available in the literature, the most probable Li-sites were obtained from the Connolly surface of the Li-poor phase and the lowest structure energy was then used to compute Bader charges and Madelung fields. For the LiFeSO 4 F triplite and the Li 2 FeP 2 O 7 phases in which Li/ M intermixing occurs [16] , [29] , averaged formal charges were considered (for example, 50% Li + and 50% Fe 2+ resulting in (Li/Fe) 1.5+ ). For the specific case of the LiFeSO 4 F triplite, the 11-ordered structures proposed in the recent work by Ben Yahia et al. [12] were considered to access average values of the Madelung fields in Figs 3 and 4 . These ordered structures present different local orders (that is, different distributions of the Li and Fe ions on the equivalent cationic sites I and II), which correspond to different connection modes between consecutive FeO 4 F 2 octahedra (edge or corner sharing). As shown in Supplementary Fig. 1 , this leads to Fe-Bader charges varying from 1.47 to 1.50 and DFT-computed cell voltages varying from 3.9 to 5.0 V ref. 12 , thus highlighting the challenge for periodic DFT calculations to accurately predict the potential of disordered materials. DFT bader charge calculations Bader charges were computed with the plane-wave DFT VASP code (Vienna Ab initio Simulation Package) [34] , [35] using the AIM atom in molecule theory implemented in the Henkelman programme [36] , [37] . Prior to charge analysis, spin-polarized DFT+U calculations were performed using the rotationally invariant Dudarev method [25] within the generalized gradient approximation with PBE functional to describe electron exchange and correlation [38] . The effective Hubbard corrections were taken from the literature for the iron ( U eff =4.0 eV) and cobalt ( U eff =5.0 eV) d -electrons [12] , [39] . A plane-wave cut-off of 600 eV was used to define the basis set, with well-converged k-point sampling for each compound. How to cite this article: Saubanère, M. et al. An intuitive and efficient method for cell voltage prediction of lithium and sodium-ion batteries. Nat. Commun. 5:5559 doi: 10.1038/ncomms6559 (2014).